Chemotactic antiviral cytokines promote infectious apical entry of human adenovirus into polarized epithelial cells Mucosal epithelia provide strong barriers against pathogens. For instance, the outward facing apical membrane of polarized epithelial cells lacks receptors for agents, such as hepatitis C virus, herpesvirus, reovirus, poliovirus or adenovirus. In addition, macrophages eliminate pathogens from the luminal space. Here we show that human adenovirus type 5 engages an antiviral immune response to enter polarized epithelial cells. Blood-derived macrophages co-cultured apically on polarized epithelial cells facilitate epithelial infection. Infection also occurs in the absence of macrophages, if virus-conditioned macrophage-medium containing the chemotactic cytokine CXCL8 (interleukin-8), or recombinant CXCL8 are present. In polarized cells, CXCL8 activates a Src-family tyrosine kinase via the apical CXCR1 and CXCR2 receptors. This activation process relocates the viral co-receptor ανβ3 integrin to the apical surface, and enables apical binding and infection with adenovirus depending on the primary adenovirus receptor CAR. This paradigm may explain how other mucosal pathogens enter epithelial cells. The airway epithelium is both a barrier and early detector for viruses. It involves a cohesive network of polarized cells and restricts the flux of fluids, ions and pathogens into and out of the respiratory organs. An increasing number of pathogenic human viruses are found to be transmitted between mucosal epithelia of individuals, including human immune deficiency virus HIV, influenza virus, enteroviruses, hepatitis A, B, C and E viruses, poxviruses and also human adenoviruses [1] , [2] . Adenoviruses are an environmental risk factor outnumbering the ubiquitous enteroviruses in surface waters [3] . Of the 55 human adenovirus types known today ( http://www.vmri.hu/~harrach/AdVtaxlong.htm ), more than one third is associated with disease. Fatal cases of adenovirus infections are mostly due to T-lymphocyte deficiencies and occur in immunosuppressed patients [4] . In normal individuals, respiratory epithelial cells are initial sites for infection, although the underlying mechanisms are unknown. This leads to respiratory disease, gastroenteritis, acute haemorrhagic cystitis, meningoencephalitis and conjunctivitis [5] , [6] , [7] . Epithelial cells adhere to each other at cell junctions, which are formed by cadherins, claudins, occludins and nectins and also immunoglobulin superfamily proteins, such as CAR (coxsackievirus-adenovirus receptor) and junction adhesion molecule (JAM [8] ). Yet, the junctions are dynamic and allow the passage of immune cells between epithelial cells. This supports inflammatory responses [9] , and somehow lays receptors open for viruses like polio, herpes, adeno, coxsackie and reovirus discussed in [10] . As the intact epithelium is resistant to infection, it has remained unknown how viruses cross epithelial barriers. Some pathogens are known to affect junctional integrity, as for instance, enteropathogenic Escherichia coli , or the extracellular human gastric bacteria Helicobacter pylori , which disrupt transepithelial resistance and retarget β1 integrin to the apical surface. Activated β1 integrin adheres to bacteria and then triggers the injection of effectors into epithelial cells, which induces proinflammatory host genes and the release of cytokines, such as interleukin-8 (CXCL8) or tumour necrosis factor-alpha (TNF-α). This, in turn, attracts and stimulates immune cells to infiltrate mucosa and eventually destroy tissue integrity reviewed in ref. 11 . Viruses do not appear to drastically affect junctional integrity. Instead, some viruses directly bind to apical receptors. For example, coxsackievirus B, a picornavirus, attaches to CD55, which triggers a signalling cascade leading to virus attachment to the tight junction protein CAR (coxsackievirus B adenovirus receptor) and infectious virus entry [12] . Similarly, the severe acute respiratory syndrome SARS coronavirus adheres to the human angiotensin converting enzyme 2 on the apical membrane of airway epithelial cells, and infects cells by receptor-mediated endocytosis [13] . Likewise, sialic acid-binding viruses, such as influenza virus, polyomavirus, rotavirus or reovirus attach to the apical side of polarized epithelial cells, although the infectious uptake mechanisms are unknown [14] . Here we provide evidence for a novel mechanism of epithelial infection, namely the stimulation of virus entry by virus-induced cytokines from immune cells. Our findings may shed light on how other pathogens enter cells. Macrophages enhance apical Ad5 infection of epithelial cells CAR localizes to the basolateral domain and tight junctions and ανβ3/5 integrins to the basal membrane of polarized airway epithelial cells, which precludes apical Ad2/5 (adenovirus type 2 and 5) binding and infection [15] , [16] . We validated this observation with two different human lung epithelial cell lines, bronchial epithelial 16HBE14o cells and alveolar type II epithelial A549 cells. When grown to confluent monolayers on transwell filters and inoculated with a non-replicating adenovirus reporter, which expresses murine interleukin (IL)-2 (Ad5-muIL2, muIL2 expression is hereafter referred to as infection) [17] , both cell types were poorly infected from the apical side, but were strongly infected from the basolateral side yielding infection levels of 20–40% of nonpolarized cell infections ( Fig. 1a ). Both cell lines expressed CAR, ανβ3- and ανβ5-integrins ( Fig. 1b ). Opening up the cell–cell contacts with EDTA significantly increased apical infection ( Fig. 1a ), consistent with results from earlier treatments of polarized cells with the divalent cation chelator ethylene-glycol-tetraacetic-acid (EGTA) [16] . These results were confirmed by green fluorescent protein (GFP) expression analyses from a replication-defective Ad5-eGFP in 16HBE14o cells ( Supplementary Fig. S1 ). 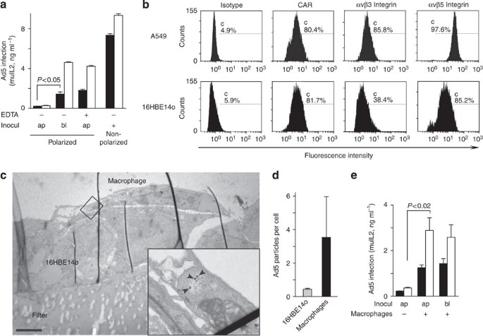Figure 1: Macrophages facilitate apical adenovirus infection. (a) Adenovirus infection of polarized epithelial cells. Polarized or subconfluent 16HBE14o (black bars) or A549 cells (open bars) were inoculated (inocul) with Ad5 expressing murine IL-2 (muIL2) for 20 h from the apical (ap) or the basal (bl) side with or without previous treatment with 20 mM EDTA for 2 min. Infection was measured by determining muIL2 levels in the supernatants using ELISA. Data represent mean of triplicates and s.e.m.; statistical relevance (P-value) was determined by Student'st-test. (b) Ad2/5 receptors CAR and ανβ3 and ανβ5 integrins are expressed on epithelial A549 and 16HBE14o cells, indicated by flow cytometry. The numbers indicate the % cells with signals larger than the threshold values (grey lines). Threshold values were defined by the isotype controls. (c) Transmission electron microscopy of 16HBE114o monolayer on transwell filter with apically added macrophages. Arrowheads indicate viral particles. The inset enlarges an area of interest. Scale bar, 5 μm. (d) Quantification of total viral particles in macropages (n=5) and epithelial cells (n=17). (e) Apical infection on addition of macrophages. Polarized 16HBE14o were infected with Ad5-muIL2 from the apical side in presence or absence of macrophages, or from the basal side for 20 or 30 h (black bars and open ars, respectively). Experiments were carried out in triplicates. Error bars represent s.e.m. values, andP-values are from Student'st-tests. Figure 1: Macrophages facilitate apical adenovirus infection. ( a ) Adenovirus infection of polarized epithelial cells. Polarized or subconfluent 16HBE14o (black bars) or A549 cells (open bars) were inoculated (inocul) with Ad5 expressing murine IL-2 (muIL2) for 20 h from the apical (ap) or the basal (bl) side with or without previous treatment with 20 mM EDTA for 2 min. Infection was measured by determining muIL2 levels in the supernatants using ELISA. Data represent mean of triplicates and s.e.m. ; statistical relevance ( P -value) was determined by Student's t -test. ( b ) Ad2/5 receptors CAR and ανβ3 and ανβ5 integrins are expressed on epithelial A549 and 16HBE14o cells, indicated by flow cytometry. The numbers indicate the % cells with signals larger than the threshold values (grey lines). Threshold values were defined by the isotype controls. ( c ) Transmission electron microscopy of 16HBE114o monolayer on transwell filter with apically added macrophages. Arrowheads indicate viral particles. The inset enlarges an area of interest. Scale bar, 5 μm. ( d ) Quantification of total viral particles in macropages ( n =5) and epithelial cells ( n =17). ( e ) Apical infection on addition of macrophages. Polarized 16HBE14o were infected with Ad5-muIL2 from the apical side in presence or absence of macrophages, or from the basal side for 20 or 30 h (black bars and open ars, respectively). Experiments were carried out in triplicates. Error bars represent s.e.m. values, and P -values are from Student's t -tests. Full size image We next assessed whether macrophages have an impact on adenovirus infection of epithelial cells. Isolated human peripheral blood mononuclear cells (PBMC)-derived macrophages could not be infected with Ad5-muIL2 up to 45 h postinfection (pi), unlike 16HBE14o cells ( Supplementary Fig. S2a ). As expected, PBMC-derived macrophages did not express the Ad2/5 attachment receptor CAR, and had moderate levels of ανβ3/5 integrins on their surface ( Supplementary Fig. S2b [18] ). To mimic the natural situation of macrophage-controlled mucosal epithelia, we seeded macrophages onto the apical side of polarized 16HBE14o monolayers and allowed attachment for 24 h. Transmission electron microscopy of macrophage and 16HBE14o co-cultures showed intact epithelial monolayers with macrophages attached to the apical membranes ( Fig. 1c ). On apical inoculation of co-cultures with Ad5 wildtype for 1 h, virions could be readily detected in vesicular structures of macrophages and to a much lower degree in epithelial cells ( Fig. 1c,d ). Epithelial cells cultured without macrophages contained no detectable virus particles (not shown). When co-cultures were inoculated with Ad5-muIL2 for 20 or 30 h, we detected no significant differences between apical or basolateral inoculations, whereas polarized epithelial cells without macrophages were not infected by apical inoculation ( Fig. 1e ). These data indicate a crucial role for macrophages in Ad5 infection of epithelial layers consisting of macrophages and epithelial cells. Apical Ad5 infection mediated by conditioned medium Macrophage-mediated apical infection depends either on direct interactions of macrophages with epithelial cells, or on messengers secreted from macrophages, such as cytokines. We tested whether the supernatant from macrophages inoculated with adenovirus, the so-called conditioned medium (CM), was sufficient to increase the Ad5-muIL2 infection of polarized epithelial cells. PBMC-derived human macrophages were inoculated with Ad2 for 4 h; the medium was collected and cleared by centrifugation and added to polarized 16HBE14o cells for 4 h, followed by apical inoculation with Ad5-muIL2 for 20 or 30 h ( Fig. 2a ). Stimulation of polarized cells with CM led to strong increase of apical infection compared with non-stimulated cells ( Fig. 2b ). Although we observed variations of CM potencies between macrophages from different blood donors, the typical increase of viral infection was 8- to 12-fold. In all instances, the maximal stimulation of apical infection was obtained at 4–8 h post stimulation ( Fig. 2c ). Interestingly, the infection stimulation was much stronger, if CM was applied apically than basolaterally, and was only marginally increased by simultaneous addition to both apical and the basal domains compared with apical stimulation ( Fig. 2d ). Importantly, the CM did not lose its potency by previous centrifugation under conditions, which completely pelleted viral particles ( Supplementary Fig. S3a ). Heat inactivation of CM at 75 °C for 15 min reduced the stimulatory activity to almost background levels, suggesting that the heat-sensitive factor(s) were responsible for the infection-stimulating effects ( Supplementary Fig. S3b ). Taken together, the data suggest that adenovirus-inoculated macrophages condition the medium with heat sensitive agents, which act on the epithelial cells from the apical side and enhance apical adenovirus infection. 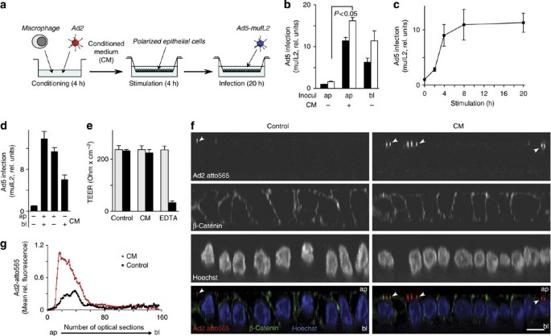Figure 2: Conditioned medium from Ad-inoculated macrophages is sufficient to facilitate apical Ad5 infection. (a) Scheme for standardized CM production and epithelial cell stimulation. Macrophages were incubated with Ad2 at 37 °C for 4 h. Supernatant CM was centrifuged at 16,000gat 4 °C for 15 min. Aliquots were stored at −20 °C until use. Polarized epithelial cells were stimulated with CM from the apical side (unless stated otherwise) at 37 °C for 4 h, followed by apical infection with Ad5-muIL2 for 20 h. (b) Apical infection on stimulation with CM. Polarized 16HBE14o were stimulated with CM for 4 h or left untreated, and infected from the apical (ap) or basal (bl) side with Ad5-muIL2 for 20 or 30 h (black and open bars, respectively). Levels of muIL2 in the supernatant were determined by ELISA and relative values obtained by normalization against apical infection for 20 h. Data represent means of triplicates and s.e.m.;P-value was determined by Student'st-test. (c) Time course of CM stimulation. Polarized 16HBE14o were stimulated with CM for 2–20 h, and infected with Ad5-muIL2 for 20 h. Infection was normalized against time point 0. Experiments were carried out in triplicates. Error bars represent s.e.m. values. (d) Apical stimulation with CM is more efficient than basal stimulation. Polarized 16HBE14o cells were stimulated with CM apically (ap), basally (bl) or both for 4 h and infected with Ad5-muIL2 for 20 h. Infection was normalized against non-treated control. Experiments were carried out in triplicates. Error bars represent s.e.m. values. (e) Impact of CM stimulation on the integrity of polarized 16HBE14o cells. TEER was determined before (0 h, control, grey bars) and after (4 h) treatment with CM or 20 mM EDTA (black bars). Data represent means of triplicates and s.e.m. (f) Enhanced apical binding of adenovirus on CM stimulation. Polarized 16HBE14o cells were treated with control medium or CM, and atto565-labelled Ad2 was cold-bound to the apical side. Samples were stained for the basolateral marker β-catenin and nuclei (Hoechst). Z-projections of confocal stacks with sections spaced by 0.19 μm are shown. Bound virions are indicated by white arrow heads. Scale bar, 10 μm. (g) Quantification of images shown in panel f. The mean relative fluorescence of Ad2-atto565 from stacks with a surface area of 246.5 μm2was plotted from the apical to the basal sides. Figure 2: Conditioned medium from Ad-inoculated macrophages is sufficient to facilitate apical Ad5 infection. ( a ) Scheme for standardized CM production and epithelial cell stimulation. Macrophages were incubated with Ad2 at 37 °C for 4 h. Supernatant CM was centrifuged at 16,000 g at 4 °C for 15 min. Aliquots were stored at −20 °C until use. Polarized epithelial cells were stimulated with CM from the apical side (unless stated otherwise) at 37 °C for 4 h, followed by apical infection with Ad5-muIL2 for 20 h. ( b ) Apical infection on stimulation with CM. Polarized 16HBE14o were stimulated with CM for 4 h or left untreated, and infected from the apical (ap) or basal (bl) side with Ad5-muIL2 for 20 or 30 h (black and open bars, respectively). Levels of muIL2 in the supernatant were determined by ELISA and relative values obtained by normalization against apical infection for 20 h. Data represent means of triplicates and s.e.m. ; P -value was determined by Student's t -test. ( c ) Time course of CM stimulation. Polarized 16HBE14o were stimulated with CM for 2–20 h, and infected with Ad5-muIL2 for 20 h. Infection was normalized against time point 0. Experiments were carried out in triplicates. Error bars represent s.e.m. values. ( d ) Apical stimulation with CM is more efficient than basal stimulation. Polarized 16HBE14o cells were stimulated with CM apically (ap), basally (bl) or both for 4 h and infected with Ad5-muIL2 for 20 h. Infection was normalized against non-treated control. Experiments were carried out in triplicates. Error bars represent s.e.m. values. ( e ) Impact of CM stimulation on the integrity of polarized 16HBE14o cells. TEER was determined before (0 h, control, grey bars) and after (4 h) treatment with CM or 20 mM EDTA (black bars). Data represent means of triplicates and s.e.m. ( f ) Enhanced apical binding of adenovirus on CM stimulation. Polarized 16HBE14o cells were treated with control medium or CM, and atto565-labelled Ad2 was cold-bound to the apical side. Samples were stained for the basolateral marker β-catenin and nuclei (Hoechst). Z-projections of confocal stacks with sections spaced by 0.19 μm are shown. Bound virions are indicated by white arrow heads. Scale bar, 10 μm. ( g ) Quantification of images shown in panel f. The mean relative fluorescence of Ad2-atto565 from stacks with a surface area of 246.5 μm 2 was plotted from the apical to the basal sides. Full size image CM enhances apical binding of Ad2/5 We measured the trans-epithelial electrical resistance (TEER) or diffusion rate of 10 kDa dextran-fluorescein isothiocyanate (FITC) across the epithelial layer. Treatment of polarized 16HBE14o cells with CM or control macrophage supernatant did not indicate any impairment of epithelial integrity, whereas EDTA treatment drastically reduced TEER ( Fig. 2e ), and increased the apparent permeability of 10 kDa FITC-dextran (50 μg ml −1 apically added for 30 min) to 9.7×10 −3 cm −2 s −1 compared with 2.5×10 −6 cm −2 s −1 in control or 0.5×10 −6 cm −2 s −1 in CM-treated cells. In a binding assay, we next analysed the localization of atto565-labelled Ad2 added to polarized 16HBE14o cells by incubation at 4 °C. Side projections of confocal fluorescence microscopy z-stacks showed an increased apical localization of Ad2-atto565 on CM-treated cells compared with cells treated with control macrophage supernatant ( Fig. 2f,g ). We did not detect viral particles in basolateral areas, or within cells, suggesting that the epithelial layers were intact. We conclude that enhanced apical infection on CM treatment is not due to disrupted junctions, but rather results from changes in the apical membrane domain composition allowing for virus attachment. CXCL8 mediates apical adenovirus infection Adenoviruses are known to trigger the secretion of cytokines from macrophages, which coordinate a concerted antiviral immune response [19] . To identify cytokines in the infection stimulating CM, we performed a BioPlex assay including 12 different cytokines with known effects on epithelial layers. At 4 h after inoculation of macrophages with adenovirus, we detected IL-6, CXCL8, IL-10 and TNF-α in the supernatant, and at 8 h, interferon (IFN)-γ was also detected, but IL-10 was no longer detected ( Supplementary Table S1 ). We did not detect IL-1β, IL-4, IL-12/p70, IL-13, IL-15, IL-17 or IFN-α2, suggesting that these cytokines have no decisive role in stimulation of epithelial infection. The treatment of polarized 16HBE14o cells with recombinant human CXCL8 (CXCL8), however, boosted apical infection in a dose-dependent manner, although not to the full extent as CM. Recombinant human IFN-gamma (IFN-γ) had no infection-supporting impact ( Fig. 3a ), although it increased the expression of HLA-1 (MHC-I) epitopes on A549 cells (data not shown). The depletion of CXCL8 from CM with a neutralizing antibody, however, significantly reduced the stimulation of apical infection, whereas depletion of IL-10 did not ( Fig. 3b ). These data suggest an important role of CXCL8 in stimulating apical adenovirus infection, although it did not account for the full stimulation by CM. This conclusion was corroborated by the finding that blocking of the CXCL8 receptors, CXCR1 and CXCR2, with neutralizing antibodies before stimulation with CM reduced CM-mediated infection to a significant extent, yet not completely ( Fig. 3c ). Neutralization of both receptors together did not have additive effects, suggesting a co-dependency of receptor function by heterodimerization, as earlier reviewed in ref. 20 . 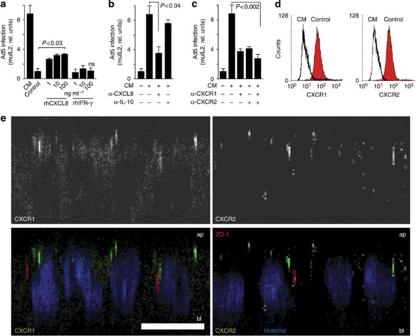Figure 3: CXCL8 is an infection stimulating component of CM. (a) Recombinant human CXCL8 boosts apical infection with adenovirus. Polarized 16HBE14o cells were treated with CM, CXCL8 or IFN-γ at indicated concentrations for 4 h, or left untreated prior to apical infection with Ad5-muIL2 for 20 h. Infection was normalized against non-treated controls. Data represent means of triplicates and s.e.m.;P-value was determined by Student'st-test. (b) Neutralizing antibody against CXCL8 significantly diminishes apical infection on CM stimulation. CM was incubated with neutralizing antibodies against CXCL8 or IL-10 before stimulation of polarized 16HBE14o cells or left untreated. Apical infection with Ad5-muIL2 was for 20 h, and normalization against non-treated controls. Experiments were carried out in triplicates. Error bars represent s.e.m. values, andP-values are from Student'st-tests. (c) Neutralizing antibodies against CXCL8 receptors CXCR1 and CXCR2 significantly reduce apical infection on CM stimulation. Polarized 16HBE14o cells were incubated with neutralizing antibodies against CXCR1, CXCR2 alone and both together before CM stimulation. Cells were infected apically with Ad5-muIL2 and infection was normalized against untreated control. Experiments were carried out in triplicates. Error bars represent s.e.m. values, andP-values are from Student'st-tests. (d) CXCR1 and CXCR2 are rapidly activated on CM stimulation, as indicated by reduction from the cell surface. Surface expressions of CXCR1 and CXCR2 were determined by flow cytometry in control 16HBE14o cells or 16HBE14o cells 10 min after stimulation with CM. (e) CXCR1 and CXCR2 are localized on the apical surface of polarized 16HBE14o cells. Polarized 16HBE14o cells were stained for CXCR1 or CXCR2, and ZO-1. Nuclei were stained with Hoechst. Z-projections of confocal stacks are shown. Scale bar, 10 μm. Figure 3: CXCL8 is an infection stimulating component of CM. ( a ) Recombinant human CXCL8 boosts apical infection with adenovirus. Polarized 16HBE14o cells were treated with CM, CXCL8 or IFN-γ at indicated concentrations for 4 h, or left untreated prior to apical infection with Ad5-muIL2 for 20 h. Infection was normalized against non-treated controls. Data represent means of triplicates and s.e.m. ; P -value was determined by Student's t -test. ( b ) Neutralizing antibody against CXCL8 significantly diminishes apical infection on CM stimulation. CM was incubated with neutralizing antibodies against CXCL8 or IL-10 before stimulation of polarized 16HBE14o cells or left untreated. Apical infection with Ad5-muIL2 was for 20 h, and normalization against non-treated controls. Experiments were carried out in triplicates. Error bars represent s.e.m. values, and P -values are from Student's t -tests. ( c ) Neutralizing antibodies against CXCL8 receptors CXCR1 and CXCR2 significantly reduce apical infection on CM stimulation. Polarized 16HBE14o cells were incubated with neutralizing antibodies against CXCR1, CXCR2 alone and both together before CM stimulation. Cells were infected apically with Ad5-muIL2 and infection was normalized against untreated control. Experiments were carried out in triplicates. Error bars represent s.e.m. values, and P -values are from Student's t -tests. ( d ) CXCR1 and CXCR2 are rapidly activated on CM stimulation, as indicated by reduction from the cell surface. Surface expressions of CXCR1 and CXCR2 were determined by flow cytometry in control 16HBE14o cells or 16HBE14o cells 10 min after stimulation with CM. ( e ) CXCR1 and CXCR2 are localized on the apical surface of polarized 16HBE14o cells. Polarized 16HBE14o cells were stained for CXCR1 or CXCR2, and ZO-1. Nuclei were stained with Hoechst. Z-projections of confocal stacks are shown. Scale bar, 10 μm. Full size image CXCR1 and CXCR2 are known to be internalized on ligand activation [21] , which initiates CXCL8 signalling [22] . We found that CM-stimulated polarized epithelial cells efficiently internalized both receptors within 10 min, which is consistent with a high degree of activation ( Fig. 3d ). Interestingly, both CXCR1 and CXCR2 were found on the apical side of polarized 16HBE14o cells by confocal imaging ( Fig. 3e ), supporting the finding that apical application of CM did stimulate infection of 16HBE14o cells ( Fig. 2d ). CM and CXCL8 induce apical localization of ανβ3 integrin Our earlier results indicated that CM did not affect the integrity of the epithelial layer excluding the possibility that receptors become accessible to apical virus particles by loosened cell–cell contact areas. We next tested whether integrin receptors were expressed on the apical surface of CM-stimulated polarized epithelial cells. Flow cytometry measurements indicated that both CAR and ανβ5-integrin total surface expression levels did not change on CM stimulation while the expression of ανβ3 integrin was slightly decreased ( Fig. 4a ). 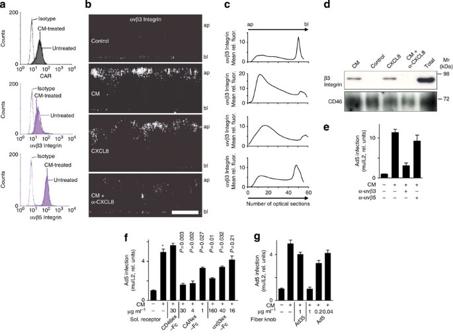Figure 4: CXCL8 is responsible for CM-induced apical translocation of ανβ3 integrin. (a) Total surface expression of adenovirus receptors CAR, ανβ3 and ανβ5 integrins determined by flow cytometry in untreated cells (black line) or after CM stimulation of confluent A549 cells for 4 h (black line, gray filled). IgG isotype control is shown in gray line. (b,c) CM and CXCL8 relocate ανβ3 integrin to the apical side. Polarized A549 cells were stimulated with CM, CXCL8 or CM incubated with neutralizing antibody against CXCL8 before stimulation. Cells were stained for ανβ3 integrin and confocal stacks were recorded. Z-projections of the stacks are shown inb. Scale bar, 15 μm. (c) Shows quantification of the mean relative fluorescence for each section of the stacks shown inb, covering an area of 246.5 μm2, plotted from the apical (ap) to the basal (bl) sections. (d) Polarized 16HBE14o cells were stimulated with CM, CXCL8 or CM incubated with neutralizing antibody against CXCL8 before stimulation. Apical cell surface was biotinylated, and biotinylated proteins were pulled down with neutravidin from cell lysates. Aliquots of biotinylated samples and total cell lysate were probed for β3 integrin and CD46 on a western blot. (e) Polarized 16HBE14o cells were stimulated with CM for 4 h or left untreated. Neutralizing antibodies against ανβ3 or ανβ5 integrins were added for the last hour. Cells were apically infected with Ad5-muIL2 for 20 h. Graph shows normalized infection compared with untreated control. Data represent means of triplicates and s.e.m. (f) Competition assay with soluble forms of Fc-tagged CAR (CARex-Fc) and αvβ3 integrin (αvβ3ex-Fc) with soluble CD46 (CD46ex-Fc) as control. Polarized 16HBE14o cells were stimulated with CM for 4 h or left untreated. Soluble virus receptors were added from the apical side and incubated at 4 °C for 1 h. Cells were apically infected with Ad5-muIL2 for 20 h. Graph shows normalized infection compared with untreated control. Data represent means of triplicates and s.e.m. withP-values from Studentst-tests relative to data indicated by* . (g) Competition assay with soluble forms of Ad5 fibre knob and Ad35 fibre knob as control. Assay was performed as described for (f). Figure 4: CXCL8 is responsible for CM-induced apical translocation of ανβ3 integrin. ( a ) Total surface expression of adenovirus receptors CAR, ανβ3 and ανβ5 integrins determined by flow cytometry in untreated cells (black line) or after CM stimulation of confluent A549 cells for 4 h (black line, gray filled). IgG isotype control is shown in gray line. ( b , c ) CM and CXCL8 relocate ανβ3 integrin to the apical side. Polarized A549 cells were stimulated with CM, CXCL8 or CM incubated with neutralizing antibody against CXCL8 before stimulation. Cells were stained for ανβ3 integrin and confocal stacks were recorded. Z-projections of the stacks are shown in b . Scale bar, 15 μm. ( c ) Shows quantification of the mean relative fluorescence for each section of the stacks shown in b , covering an area of 246.5 μm 2 , plotted from the apical (ap) to the basal (bl) sections. ( d ) Polarized 16HBE14o cells were stimulated with CM, CXCL8 or CM incubated with neutralizing antibody against CXCL8 before stimulation. Apical cell surface was biotinylated, and biotinylated proteins were pulled down with neutravidin from cell lysates. Aliquots of biotinylated samples and total cell lysate were probed for β3 integrin and CD46 on a western blot. ( e ) Polarized 16HBE14o cells were stimulated with CM for 4 h or left untreated. Neutralizing antibodies against ανβ3 or ανβ5 integrins were added for the last hour. Cells were apically infected with Ad5-muIL2 for 20 h. Graph shows normalized infection compared with untreated control. Data represent means of triplicates and s.e.m. ( f ) Competition assay with soluble forms of Fc-tagged CAR (CARex-Fc) and αvβ3 integrin (αvβ3ex-Fc) with soluble CD46 (CD46ex-Fc) as control. Polarized 16HBE14o cells were stimulated with CM for 4 h or left untreated. Soluble virus receptors were added from the apical side and incubated at 4 °C for 1 h. Cells were apically infected with Ad5-muIL2 for 20 h. Graph shows normalized infection compared with untreated control. Data represent means of triplicates and s.e.m. with P -values from Students t -tests relative to data indicated by* . ( g ) Competition assay with soluble forms of Ad5 fibre knob and Ad35 fibre knob as control. Assay was performed as described for ( f ). Full size image We examined the localization of ανβ3 and ανβ5 integrins in polarized 16HBE14o cells by confocal fluorescence microscopy. Intriguingly, side projections of z-stacks showed that ανβ3 integrin was present on the apical membranes on stimulation by CM or CXCL8 ( Fig. 4b ), whereas ανβ5 integrin remained localized to the basolateral domains ( Supplementary Fig. S4a,b ). The treatment of CM with neutralizing antibodies against CXCL8 before stimulation abrogated the apical localization of ανβ3 integrin ( Fig. 4b,c ). We confirmed these results by selective biotinylation of the apical cell surface and subsequent neutravidin pull-downs of biotinylated proteins ( Fig. 4d ). Further analysis by SDS–PAGE and western blotting identified β3 integrin as one of the biotinylated, thus apical proteins. The membrane cofactor CD46, which was reported to localize to the apical membrane compartment [23] , was also significantly biotinylated from the apical side, similar to β3 integrin ( Fig. 4d ). We next tested the functional significance of the apical localization of ανβ3 integrin on CM stimulation. Apical addition of anti-ανβ3 integrin function blocking antibodies to CM-stimulated 16HBE14o cells strongly reduced Ad5-muIL2 infection, whereas anti-ανβ5 integrin antibodies had no significant effects ( Fig. 4e ). We further confirmed the role of the receptors ανβ3 integrin and CAR in apical infection on CM stimulation with competition experiments. Soluble forms of CAR and integrin receptors added after the 4 h stimulation period were able to interfere with infection in a dose-dependent manner ( Fig. 4f ). Control soluble CD46, however, had no effect. Likewise, soluble Ad2 fibre knob inhibited infection whereas Ad35 fibre knob, which does not bind CAR, showed no effect ( Fig. 4g ). In agreement with these functional interference data, we found CAR epitopes on the apical side of CM stimulated 16HBE14o cells, distinct from the tight junction marker ZO-1 ( Supplementary Fig. S4c ). These results were in line with the co-localization of ανβ3 integrin and CAR with Ad2-atto565 particles added apically to stimulated cells (not shown). Together, the data suggest that CM or CXCL8 enhance the localization of ανβ3 integrin and CAR to the apical domain without grossly altering the overall cell surface expression of ανβ3 integrin. This enables adenovirus attachment to the apical cell surface and subsequent infection. β3 integrin localization and apical infection are Src-dependent To address the nature of apical ανβ3 integrin-mediated adenovirus infection, we tested the hypothesis that a mechanism akin to emerging focal complexes could be involved, which is also implicated in cell migration and wound healing. Focal contacts around integrins mediate cell adhesion to the extracellular matrix. They are dynamically regulated in migratory cells by tyrosine kinase signalling [24] . It is of note that the chemokine CXCL8 not only acts as an important chemo-attractant to neutrophils and initiates directed cell migration, it has also been implicated in inducing wound healing and migration of epithelial and endothelial cells [25] . CXCL8 leads to formation of focal complexes by signalling via Src/FAK and paxillin [26] . We tested whether signalling via Src and paxillin is involved in ανβ3 integrin relocalization. Serum-starved 16HBE14o cells were stimulated with either control medium (supernatant of non-inoculated macrophages), CM, CXCL8 or CXCL8 depleted CM for 10 min or 4 h. Strong induction of Src tyrosine 416 (Y416) phosphorylation could be detected in both CM and CXCL8-treated cells at 10 min or 4 h post treatment ( Fig. 5a ). Likewise, phosphorylation of paxillin on the critical tyrosine residue Y118 was induced by CM and CXCL8 at 4 h, and confirmed by immunofluorescence microscopy, which showed apical localization of pY118 paxillin ( Fig. 5b ; Supplementary Fig. S5a ). 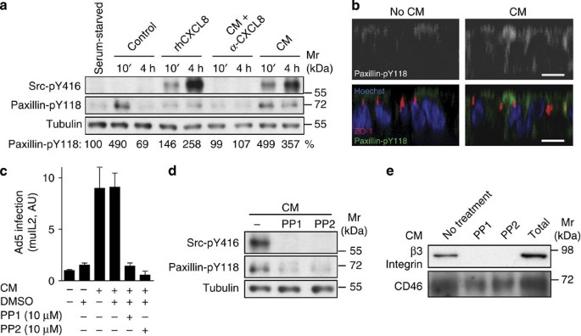Figure 5: CM-stimulated apical ανβ3 integrin localization and Ad5 infection are Src-dependent. (a) Src and paxillin are phosphorylated on CM stimulation. Confluent 16HBE14o cells were serum-starved for 24 h and subsequently stimulated for 10 min or 4 h with media containing serum (control), CM, CXCL8 or CM incubated with neutralizing antibody against CXCL8 before stimulation. Samples were analysed by western blot and probed for paxillin (phospho-Y118), Src (phospho-Y416) or tubulin. Note that there is a significant short-term signal of paxillin (phospho-Y118) in control (serum-stimulated) cells. (b) Phospho-paxillin localizes to the apical side on CM stimulation. Polarized 16HBE14o cells were stimulated with control medium and CM and stained for paxillin (phospho-Y118), ZO-1 and nuclei (Hoechst). Confocal stacks were recorded and z-projections composed. Scale bar, 10 μm. (c) Src-inhibitors PP1 and PP2 inhibit apical Ad5 infection on CM stimulation. Polarized 16HBE14o cells were treated with DMSO, PP1 and PP2 (10 μM) for 1 h or left untreated (DMSO). Subsequently, cells were stimulated with CM for 4 h, and infected with Ad5-muIL2 for 20 h. Infection was normalized against controls. Data represent mean of triplicates and s.e.m. (d) PP1 and PP2 prevent phosphorylation of Src and reduce phosphorylation of paxillin. Confluent 16HBE14o cells were serum starved for 24 h. Cells were treated with PP1 and PP2 (10 μM) for 1 h, and stimulated with CM. Aliquots of total cell lysates were analysed by western blot and probed for paxillin (phospho-Y118), Src (phospho-Y416) or tubulin. (e) Polarized 16HBE14o cells were treated with DMSO, PP1 or PP2 (10 μM) for 1 h, and subsequently stimulated with CM for 4 h. Cells were biotinylated on the apical side, lysed and biotinylated proteins were pulled down with neutravidin. Aliquots of biotinylated samples and total cell lysate were probed for β3 integrin and CD46 on a western blot. Figure 5: CM-stimulated apical ανβ3 integrin localization and Ad5 infection are Src-dependent. ( a ) Src and paxillin are phosphorylated on CM stimulation. Confluent 16HBE14o cells were serum-starved for 24 h and subsequently stimulated for 10 min or 4 h with media containing serum (control), CM, CXCL8 or CM incubated with neutralizing antibody against CXCL8 before stimulation. Samples were analysed by western blot and probed for paxillin (phospho-Y118), Src (phospho-Y416) or tubulin. Note that there is a significant short-term signal of paxillin (phospho-Y118) in control (serum-stimulated) cells. ( b ) Phospho-paxillin localizes to the apical side on CM stimulation. Polarized 16HBE14o cells were stimulated with control medium and CM and stained for paxillin (phospho-Y118), ZO-1 and nuclei (Hoechst). Confocal stacks were recorded and z-projections composed. Scale bar, 10 μm. ( c ) Src-inhibitors PP1 and PP2 inhibit apical Ad5 infection on CM stimulation. Polarized 16HBE14o cells were treated with DMSO, PP1 and PP2 (10 μM) for 1 h or left untreated (DMSO). Subsequently, cells were stimulated with CM for 4 h, and infected with Ad5-muIL2 for 20 h. Infection was normalized against controls. Data represent mean of triplicates and s.e.m. ( d ) PP1 and PP2 prevent phosphorylation of Src and reduce phosphorylation of paxillin. Confluent 16HBE14o cells were serum starved for 24 h. Cells were treated with PP1 and PP2 (10 μM) for 1 h, and stimulated with CM. Aliquots of total cell lysates were analysed by western blot and probed for paxillin (phospho-Y118), Src (phospho-Y416) or tubulin. ( e ) Polarized 16HBE14o cells were treated with DMSO, PP1 or PP2 (10 μM) for 1 h, and subsequently stimulated with CM for 4 h. Cells were biotinylated on the apical side, lysed and biotinylated proteins were pulled down with neutravidin. Aliquots of biotinylated samples and total cell lysate were probed for β3 integrin and CD46 on a western blot. Full size image To test whether Src family tyrosine kinases were involved in CM-mediated apical infection, we blocked Src activity with the small compounds PP1 and PP2 (ref. 27 ). The treatment of polarized 16HBE14o cells with PP1 and PP2 before CM stimulation had no effects on TEER ( Supplementary Fig. S5b ). However, both compounds blocked CM-mediated infection at 10 μM concentrations ( Fig. 5c ). Western blot analysis showed that PP1 and PP2 not only inhibited Src and pY118 paxillin phosphorylation, but also blocked the apical localization of ανβ3 integrin in CM-stimulated 16HBE14o cells ( Fig. 5d,e ). The data suggest that Src controls β3 integrin redistribution and apical adenovirus infection ( Fig. 6 ). 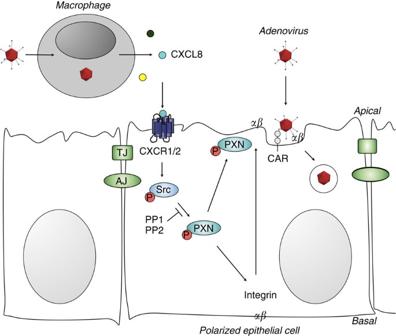Figure 6: Schematic model for apical adenovirus infection route. Adenovirus particles are taken up by apical macrophages, which subsequently release cytokines, such as CXCL8. CXCL8 triggers a signalling cascade in epithelial cells by activating its receptors CXCR1 and CXCR2. In the course of this signalling, Src and PXN are phosphorylated, and this is required for apical localization of phosphorylated paxillin and ανβ3 integrin. Together with apically localized CAR this allows apical binding of adenovirus and infection. AJ, adherens junction; CXCR, CXC chemokine receptor; PP1/2, Src tyrosine kinase inhibitors; PXN, paxillin; Src, Sarcoma tyrosine kinase; TJ, tight junction. Figure 6: Schematic model for apical adenovirus infection route. Adenovirus particles are taken up by apical macrophages, which subsequently release cytokines, such as CXCL8. CXCL8 triggers a signalling cascade in epithelial cells by activating its receptors CXCR1 and CXCR2. In the course of this signalling, Src and PXN are phosphorylated, and this is required for apical localization of phosphorylated paxillin and ανβ3 integrin. Together with apically localized CAR this allows apical binding of adenovirus and infection. AJ, adherens junction; CXCR, CXC chemokine receptor; PP1/2, Src tyrosine kinase inhibitors; PXN, paxillin; Src, Sarcoma tyrosine kinase; TJ, tight junction. Full size image Cells of the innate immune system, including macrophages and dendritic cells control the inflammatory response by interacting with epithelial cells. Alveolar macrophages are sensors for infection and detect adenoviruses in the airway lumen [28] . On contact with viruses, they undergo rapid activation and secrete pro-inflammatory cytokines, such as IL-6, CXCL8 and TNF-α [29] , [30] . This boosts the antiviral response, attracts leukocytes to the site of infection and critically contributes to mounting adaptive immune responses against the virus. However, activated macrophages also trigger acute lung injury and thereby exacerbate viral infection [2] . Our study here identifies a mechanism, by which activated macrophages increase viral infection of polarized epithelial cells. We show that macrophages co-cultured with polarized epithelial cells on the lumenal side take up virus particles and secrete cytokines, which enhance infection of the epithelial cells with adenovirus. This cytokine response does not impair the barrier function of the epithelial cells and does not require the presence of macrophages, suggesting that the infection route depends on a viral receptor in the apical epithelial membrane rather than direct transmission of viral particles from macrophages to epithelial cells, for example, a 'Trojan-horse' mechanism as proposed for measles virus [31] . Cytokine mRNAs and proteins, including IL-6, CXCL8 are induced in response to adenovirus infection in several cell lines and also in vivo [32] . For example, CXCL8 was elevated in bronchial alveolar lavage fluid of macaque monkeys on inoculation of an adenovirus vector encoding the cystic fibrosis gene, and enhanced tissue toxicity [33] , or the proinflammatory cytokines TNF-α, IL-6 and CXCL8 were strongly induced in children with symptomatic human adenovirus viremia after stem cell transplantation [34] . In epithelial cells, the genomes of adenoviruses counter the antiviral effects of the cytokines by expressing early region three genes, and thereby downregulate cytokine mRNAs and protein levels [35] . In macrophages, however, the levels of viral gene expression are low, possibly due to inefficient delivery of viral genomes to the nucleus (reviewed in 28). Hence, we readily found four of the twelve tested cytokines in virus-conditioned macrophage medium, that is, CXCL8, IL-6, TNF-α and IFN-γ. While IFN-γ had no effect, recombinant chemokine CXCL8 and activation of its receptors CXCR1/2 strongly enhanced the infection, although not to the full extent as CM. CM was more potent than isolated cytokines in stimulating infection of nonpolarized cells, but the specific components of CM responsible for these effects are unknown. In contrast, the CXCL8 ligand–receptor pair is best known for its angiogenic and neutrophil chemotactic properties [36] . CXCL8-driven chemotaxis can be elicited in many cell types expressing CXCR1/2. It has an important role in fibroblast-mediated wound healing [37] , the formation of tumour metastases [38] , and neutrophile chemotaxis [37] . Chemotaxis forms and dismantles focal complexes and adhesions, and dynamically modulates anchorage of cells to the extracellular matrix. Anchorage involves ανβ3 integrin, initially in the leading edge of migrating cells [39] . Intriguingly, CXCL8 enhancement of apical adenovirus infection required the induced localization of ανβ3 integrin in the apical plasma membrane of the polarized epithelial cells, as indicated by neutralizing antibodies or soluble ανβ3 integrin competition, which also blocks infection of nonpolarized cells (CJ Burckhardt, M Suomalainen, P Schoenenberger, K.B., S.H. and U.F.G., unpublished results). ανβ3 integrin has an important role in viral infections, where it serves as an affinity-regulated co-receptor by binding to a 50-amino-acid RGD stretch of the adenoviral capsid protein penton base [40] , [41] , and also critically contributes to HIV infection of adherent macrophages [42] . Chemotaxis critically involves the non-receptor tyrosine kinase family Src and paxillin, a pivotal signalling integrator and scaffolding protein [24] , [39] , [43] . Src directly binds the cytoplasmic tail of β3 integrin and is activated by ανβ3 integrin [44] , [45] , which might induce a positive feedback loop for integrin and Src activation. Activated Src undergoes autophosphorylation on tyrosine 416 inducing a complex with focal adhesion kinase, which then phosphorylates paxillin on its critical tyrosine residue 118 (refs 39 , 46 , 47 , 48 ). The stimulation of polarized epithelial cells with conditioned medium leads to phosphorylation of a Src-family kinase at Y416 and paxillin at Y118, indicating that this pathway is activated. This pathway is crucial for infection, because inhibition of Src family tyrosine kinases with PP1 and PP2 leads to loss of Src and paxillin phosphorylation, failure of ανβ3 integrin relocalization, and abrogated the infection stimulation. Paxillin may function in ανβ3 trafficking or as a component of a retention mechanism holding ανβ3 on the apical membrane on stimulation. Collectively, the data strongly suggest that the conditioned macrophage medium enhances apical infection by the formation of focal contacts and adhesion sites that are normally found in migratory cells. In addition to prominent apical localization of focal contact proteins, macrophage-conditioned medium also enhanced the localization of CAR on the apical membrane. CAR has been reported to potentially co-localize with ανβ3 integrin in lipid-rich membrane patches [49] , [50] . It critically supports infection, as indicated by soluble CAR and viral fibre knob competition experiments. In normal polarized epithelial cells, CAR is restricted to the baso-lateral domain and tight junctions by an intracellular trafficking mechanism involving the clathrin-adaptor AP1B [51] . Whether CAR is specifically delivered to the apical membrane or released from tight junctions remains to be investigated. In any case, the virus makes CAR available for apical infection. In doing so, it takes advantage of antiviral functions of CAR on epithelial cells, where CAR binds JAML from neutrophils, and thereby supports the infiltration of immune cells at sites of cell injury and infection [52] . Strikingly, epithelial CAR also enhances wound-healing in mucosal tissue by activating and binding to JAML on gamma-delta T cells [53] . These cells have important roles in primary defence of epithelial barriers against infection, traumatic insults and malignancies. These cells might have pivotal roles in the defence against adenoviral infection, and if impaired contribute to the severe pathological conditions in immunocompromised individuals. Collectively, our results uncover a novel apical infection route for adenovirus. We showed that innate immune cells release CXCL8, which triggers a signalling cascade in polarized epithelial cells resembling the induction of cell migration. During this process, Src and paxillin are tyrosine phosphorylated on critical residues. The latter is recruited to the apical membrane together with ανβ3 integrin, depending on Src. In the course of this activation, the immune modulator CAR is localized to the apical membrane and becomes available for binding of virus, which together with ανβ3 integrins triggers viral uptake and infection. This infection mechanism allows viral pathogens to take advantage of immunological antiviral reactions and gain entry into a well-protected epithelium. We anticipate that other viruses whose receptors are not available for virus binding in an intact uninjured epithelium can use similar strategies to achieve entry into cells. Cell lines and viruses Human transformed embryonic retinoblast 911 cells were grown in DMEM medium (D6429, Sigma) supplemented with 10% FCS (Invitrogen), 1% L -glutamine and 1% non-essential amino acids (NEA, Sigma). Carcinoma alveolar type II A549 (ATCC) and transformed bronchial epithelial 16HBE14o cells obtained from Dr D. Gruenert, California Pacific Medical Center Research Institute, San Francisco, USA [54] , were grown in RPMI 1640 medium (R8758, Sigma) supplemented with 10% FCS, 1% L -glutamine and 1% NEA. All cells were kept at low passage number at 37 °C in a humidified chamber at 5% CO 2 . For microscopy of sub-confluent cells, cells were grown to 70% confluency on 18 mm glass cover slips (Menzel Gläser). Flow cytometry was performed with cells grown to 100% confluency in 24-well-plate format. Ad5_CMV_eGFP and Ad2 were propagated in 911 cells and isolated and Ad2 was labelled with atto565 (Atto-TEC GmbH, Ad2-atto565) as described previously [55] . Ad5_CMV_muIL2 was grown as described [17] . Virus preparations used for stimulation of macrophages were tested for possible endotoxin contaminations with Endochrome Endpoint Assay Kit (Charles River Laboratories). Endotoxin levels were below 0.003 U ml −1 . Soluble CAR and CD46 were produced as described in refs 56 , 57 . Soluble αvβ3 integrin was produced in COS cells transfected with cDNAs for αv and β3 integrins tagged with human Fc (1,222 amino acids for the mature αv–Fc fusion protein, and 948 amino acids for the β3–Fc), provided by Dr Curzio Ruegg (University of Fribourg, Switzerland). Fusion proteins were produced and purified as described [56] . Ad5 or Ad35 fibre knob proteins were produced using the Bac-to-Bac baculovirus expression system (pFastBac, Stratagene) with amino-terminal 6xhis-tag for single-step Ni-NTA-agarose affinity chromatography, followed by the recognition site for TEV protease. Fibre knobs comprised the residues 384 to 581 for Ad5 (GI: 56160559) and 126 to 323 for Ad35 (GI: 56160945). Macrophage cell culture Macrophages were differentiated from human peripheral blood monocytes as described previously [58] . In brief, peripheral blood monocytes were isolated from buffy coats (blood donation service, Zurich, Switzerland) by density gradient centrifugation on Histopaque (Sigma). PBMCs were washed intensively in PBS and resuspended in RPMI 1640 supplemented with 1% L -glutamine, 1% penicillin/streptomycin and 10% heat-inactivated human serum (blood donation service). Cells were seeded at a density of 10 7 cells ml −1 and well in a 6-well-plate (Nunc) and allowed to adhere for 4 h. Non-adherent cells were washed away and adherent cells cultured as described above. Macrophages were obtained without any additional supplements. Cells were kept at 37 °C in 5% CO 2 humidified atmosphere. Purity of differentiated cells (approximately 4×10 5 cells per 6-well dish) was assessed by flow cytometry with CD14 (BD Biosciences) as monocytes/macrophage marker and yielded in >95% positive cells. Epithelial monolayers and macrophage co-culture Establishment of epithelial monolayers and co-cultures was modified after Rothen-Rutishauser [59] . Briefly, epithelial cells were seeded onto cell culture inserts (3 μm pores, 24-well (353492) or 12-well (353292) format, BD Bioscience) and allowed to settle for 2 days. Seeding to filters occurred at 150% plastic dish confluency to compensate for reduction in adhesion area during the differentiation process of the epithelial cells at air–liquid interface. Medium was removed, cells were washed with PBS and subsequently kept at an air–liquid interface supplemented with medium only from the basal side (100 μl in 24-wells, 250 μl in 12-wells). A549 cells required 9–10 days to form a monolayer of appropriate integrity, whereas 16HBE14o could be used after 6–8 days. To obtain co-cultures, macrophages were seeded on top of epithelial cells from the apical side at a ratio of approximately 2:3, settled for 2 h, unattached cells rinsed off, and co-cultures (5–10 epithelial cells per macrophage) maintained at air–liquid interface for 24 h before use. TEER and diffusion assay Integrity of epithelial monolayers was assessed by measuring TEER and the apparent permeability (Perm app ). TEER was measured with an EVOM Volt-Ohmmeter (World Precision Instruments). To determine the diffusion rate, 50 μg ml −1 10 kD FITC-dextran (Sigma-Aldrich) was added to the apical side and cells were incubated for 30 min. Aliquots were taken from the apical and basal side and fluorescence was measured using a Safire monochomator-based microplate detection system (Tecan). The apparent permeability (Perm app ) was calculated according to the following equation: where d q /d t (μg per s) is the rate of transport, C o is the initial concentration in the apical compartment (μg ml −1 ) and A is the surface area of the filter (cm 2 ). Conditioned medium Differentiated macrophages were incubated with 0.1 μg Ad2 in 1 ml per 6-well (80% confluency) at 37 °C for indicated times. Conditioned media were removed and centrifuged at 16,000 g at 4 °C for 5 min. Supernatant of non-treated macrophages was used as control. For the ultracentrifugation control samples were centrifuged at 125,000 g for 1 h. Heat inactivation was performed at 75 °C for 15 min. Aliquots of 0.5–1 ml were stored at −20 °C until use. Infections Monolayers or co-cultures in 24-well format were used for infection studies. Cells were treated with control, CM or recombinant human cytokines as indicated. CXCL8 was obtained from R&D Systems, the IFN-γ preparation had a concentration of about 10 7 U ml −1 and was used as described [60] . For blocking experiments, CM was incubated with neutralizing antibodies (R&D Systems) 1 h before stimulation of monolayers. For drug studies, polarized epithelial cells were incubated with Src-inhibitors PP1 and PP2 (Enzo Life Sciences) for 1 h before stimulation. For competition experiments, polarized 16HBE14o cells were stimulated with CM at 37 °C for 4 h, and incubated with soluble CD46, CAR, αvβ3 integrin, Ad2 fibre knob or Ad35 fibre knob at 4 °C for 1 h. Cells were infected with 10 5 pfu per well of either Ad5_CMV_muIL2 or Ad5_CMV_eGFP reporter virus from the apical or basal side. In case of co-culture experiments, medium was changed after 8 h and infection continued for another 12 h on air–liquid interface with 100 μl of medium in the bottom chamber. In all other experiments, medium in both chambers was removed after 1 h and infection proceeded for another 19 h on air–liquid interface with 100 μl of medium in the bottom chamber. Concentration of muIL2 in the media was assessed by muIL2 ELISA according to the manufacturer's protocol (BD Biosciences). GFP-expression was visualized by confocal microscopy (CLSM (Leica SP5, Leica Microsystems)). Immunofluorescence and flow cytometry Monolayers were cultured on 12-well cell culture inserts as described above and treated with control (PBS), CM, CXCL8 or CM preincubated with anti-CXCL8 neutralizing antibodies for 4 h. Cells were fixed with 3% paraformaldehyde (PFA), quenched with 25 mM NH 4 Cl and permeabilized with 0.5% Triton X-100. Filters were quartered and incubated with the first antibody at 4 °C overnight. The following antibodies were used: mouse monoclonal anti-CAR (E1-1, culture supernatant) [56] , mouse monoclonal anti-integrin αvβ3 (1:100, clone LM609, Chemicon), mouse monoclonal anti-integrin αvβ5 (1:100, clone P1F6, Chemicon), mouse monoclonal anti-beta-catenin (1:500, clone 14, BD Transduction Laboratories), mouse monoclonal anti-occludin (1:200, clone 19, BD Transduction), mouse monoclonal anti-ZO-1 (1:200, clone 1, BD Transduction), rabbit anti-ZO-1 (1:200, ab59720, Abcam), rabbit anti-paxillin-pY118 (1:500, A00379, GenScript). Secondary antibodies (anti-mouse Alexa488, anti-mouse Alexa594, anti-mouse Cy5, anti-rabbit Alexa594; all from Molecular Probes) were incubated at 4 °C for 1 h (1:100), post-fixed with 3% PFA, and filter pieces mounted on microscopy slides. For flow cytometry, cells were detached with accutase (Sigma), blocked with 10% human serum for 1 h, and incubated with primary antibodies at 4 °C on a rotator for 2 h. Secondary antibodies were incubated at 4 °C on a rotator for 1 h. Acquisition was performed with a FACScan (Beckman Coulter FC500 Cytometer). About 10 4 cells were measured for each condition using antibody dilutions as indicated above. Binding assay Cells were grown on 12-well cell culture inserts as described above. Ad2-atto565 was allowed to bind to the cells at 4 °C for 30 min, fixed with 3% PFA, and stained for tight junction marker or receptor proteins as described above. Biotinylation assay Confluent monolayers (12-well format) were washed twice with ice-cold HBSS +/+ (Gibco) and biotinylated with 0.5 mg ml −1 biotin (Sulfo-NHS-SS-Biotin, Pierce) from the apical side at 4 °C for 30 min, followed by addition of quenching buffer (0.1 M glycine, 0.3% BSA in HBSS +/+), first to the basal side and then to both sides for 5 min on ice, washed three times with ice-cold HBSS +/+ and lysed in NP-40 lysis buffer. Biotinylated proteins were precipitated on neutravidin beads (UltraLink Immobilized NeutrAvidin Protein, Pierce), washed intensively and proteins eluted by boiling the samples in SDS–PAGE loading buffer. Samples were analysed by SDS–PAGE. SDS–PAGE and Western blotting Cell lysates were separated on 10% SDS–PAGE, transferred to Hybond-ECL PVDF 0.45 μm membrane (Amersham Biosciences) and blocked with 5% dried milk in 50 mM Tris/100 mM sodium chloride/0.1% Tween, pH 7.5 (TBST). The following antibodies were used: mouse monoclonal anti-Src-pY416 (1:1,000, clone 9A6, Millipore/Upstate), rabbit anti-paxillin-pY118 (1:1,000, A00379, GenScript), anti-beta 3 integrin (1:1,000, clone LM609, Chemicon), anti-CD46 (1:1,000, clone H294, Santa Cruz), rabbit anti-tubulin (1:2,000, T13). Antibodies were diluted in TBST/5% BSA (phospho-antibodies) or TBST/2.5% dried milk (all other antibodies). HRP-conjugated secondary antibodies were detected with ECL-Plus reagents (Amersham Biosciences). Filters were stripped with 100 mM β-mercaptoethanol, 2% SDS, and 62.5 mM Tris–HCl, pH 6.7, for 30 min at 50 °C, washed extensively with TBST, blocked with 5% dried milk, and reprobed with control or total antibody. Microscopy Confocal laser scanning microscopy was conducted with an inverted Leica SP5 microscope (Leica Microsystems) equipped with a 63x objective (oil immersion; NA, 1.4), a diode laser (405-nm excitation), an argon laser (458/476/488/496/514-nm excitation), and a helium laser (561/594/633-nm excitation). Image processing was performed using ImageJ open software ( http://rsbweb.nih.gov/nih-image/ ). Samples for transmission electron microscopy were fixed in 1.5% glutaraldehyde-2% formaldehyde in 0.1 M cacodylate buffer (pH 7.4) for 60 min, followed by postfixation in 1% OsO 4 and 1.5% potassium-ferricyanide at RT for 1 h, and staining with 3% uranylacetate over-night. Samples were dehydrated with aceton, embedded in Epon, ultrathin-sectioned and analysed in a Zeiss EM10. How to cite this article: Lütschg, V. et al . Chemotactic antiviral cytokines promote infectious apical entry of human adenovirus into polarized epithelial cells. Nat. Commun. 2:391 doi: 10.1038/ncomms1391 (2011).